Fast and ultrasensitive method for quantitating prion infectivity titre Bioassay by end-point dilution has been used for decades for routine determination of prion infectivity titre. Here we show that the new protein misfolding cyclic amplification with beads (PMCAb) technique can be used to estimate titres of the infection-specific forms of the prion protein with a higher level of precision and in 3–6 days as opposed to 2 years, when compared with the bioassay. For two hamster strains, 263 K and SSLOW, the median reactive doses determined by PCMAb (PMCAb 50 ) were found to be 10 12.8 and 10 12.2 per gram of brain tissue, which are 160- and 4,000-fold higher than the corresponding median infectious dose (ID 50 ) values measured by bioassay. The 10 2 - to 10 3 -fold differences between ID 50 and PMCAb 50 values could be due to a large excess of PMCAb-reactive prion protein seeds with little or no infectivity. Alternatively, the differences between ID 50 and PMCAb 50 could be due to higher rate of clearance of infection-specific prion protein seeds in animals versus PMCAb reactions. A well-calibrated PMCAb reaction can be an efficient and cost-effective method for the estimation of infection-specific prion protein titre. A pathognomonic hallmark of the prion diseases is the accumulation of the misfolded isoform of the prion protein (PrP Sc ). The traditional method for obtaining a quantitative estimate of prion infectivity is end-point dilution titration in animals. A suspension of the tissue or fluid of interest is diluted in tenfold serial steps, and then each dilution is inoculated into a group of animals. A dilution at which only a fraction of the inoculated animals develops clinical signs of disease or shows positive evidence of PrP Sc on immunoassay is called a 'limiting dilution'. At limiting dilution there are only one or a few infectious doses per inoculation volume. End-point dilution titres are typically expressed as the median infective dose (ID 50 ): the reciprocal of the dilution required to infect only 50% of the animals inoculated as determined by interpolation or other statistical methods. While the end-point bioassay has been the principal method for determining prion infectivity, the assay is extremely long, expensive and laborious. Moreover, the bioassay works optimally only for prion strains with incubation times well within the lifespan of the host. Alternatives to end-point titration are biochemical or immunochemical assays that assess either the presence, mass or concentration of PrP Sc (refs 1 , 2 , 3 , 4 ). However, establishing accurate quantitative relationships between PrP Sc concentration and prion titre has proven to be difficult because of the size heterogeneity of prion particles and uncertainty over whether all prion particles are equally infectious [5] , [6] , [7] . Moreover, the size distribution and physical properties of prion particles appear to vary with agent strain and host species [6] . In 2003, Weissmann and co-workers [8] introduced a scrapie cell assay that quantitatively estimates prion infectivity titres within a much shorter time frame than animal bioassay. The scrapie cell assay was shown to be capable of detecting prions in a dilution as low as 10 10 -fold of scrapie-infected brain material [9] . Moreover, in recent studies, the scrapie cell assay was adapted for detecting prions from various species [10] . Protein misfolding cyclic amplification (PMCA) propagates PrP Sc and infectivity in vitro [11] , [12] , [13] , [14] . The sensitivity of the PMCA reaction to detect prion particles exceeds that of the bioassay [15] , [16] . While PMCA has been proven for detecting and amplifying prions from a broad range of species including human, cow, sheep, cervids, mouse, hamster and others [16] , [17] , [18] , [19] , [20] , [21] , [22] , [23] , [24] , [25] , [26] , highly robust PMCA amplification has been limited to mostly rodent and rodent-adapted strains. Nevertheless, the efficiency of prion replication in PMCA was shown to mimic cross-species transmission barriers [27] , [28] , [29] or genetic susceptibility of sheep to scrapie that occurs due to prion protein polymorphisms [19] . The improvements in the PMCA assay found in PMCA with beads (PMCAb) have resulted in a much faster, more robust, sensitive and cost-efficient way of measuring PrP Sc compared with either PMCA or bioassay [29] , [30] . To illustrate the advantages of PMCAb-based end-point titration, we assessed the relative concentrations of PrP Sc in brain material of two rodent strains, 263K and SSLOW, which display very short or very long incubation times to symptomatic disease, respectively [31] . We show that using the PMCAb format PrP Sc titration can be performed in only a few days. We also observed strain-specific differences in the specific infectivity relative to PMCAb-based PrP Sc titre ranging from hundreds to thousands of PMCAb-active particles per intracranial infectious dose 50 (ic ID 50 ). End-point dilution titration using PMCAb The PMCAb amplification was initiated by 'seeding' a substrate of uninfected brain homogenate (BH) with PrP Sc . To determine the concentration of PMCAb seeds, 10% BHs prepared from 263K- or SSLOW-infected animals were diluted in tenfold serial steps, then aliquots from each dilution were used to seed serial PMCAb reactions. Up to ten independent serial PMCAb reactions were conducted for each dilution for each strain. Each PMCAb round consisted of 48 cycles, 30 min each. Three or six serial PMCAb rounds were sufficient for amplification of even the highest dilutions of 263K or SSLOW, respectively ( Fig. 1a,b ), to the level detectible by western blot. An increase in the number of PMCAb rounds did not increase the percentage of positive reactions for the most highly diluted samples illustrating that the limiting dilution was reached ( Fig. 1c ). 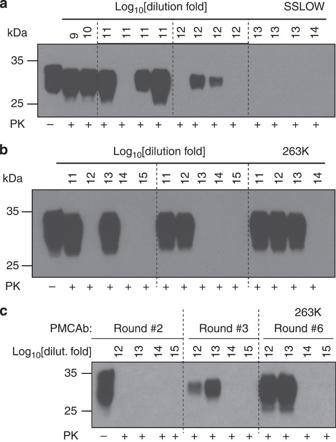Figure 1: End-point sPMCAb titration. 10% scrapie brain material from SSLOW- (a) or 263K-infected animals (b,c) were diluted in tenfold serial steps, then aliquots from each dilution were used to seed serial PMCAb reactions. Example of a western blot of serial PMCAb (sPMCAb) products amplified for six rounds is shown in plotsaandb. Panelcshows products of PMCAb reactions seeded with four dilutions and amplified for 2, 3 or 6 serial rounds. The dilutions shown for PMCAb reactions were normalized per gram of brain tissue, to correct for differences in assay volumes used for PMCAb (100 μl) and bioassay (50 μl). Figure 1: End-point sPMCAb titration. 10% scrapie brain material from SSLOW- ( a ) or 263K-infected animals ( b , c ) were diluted in tenfold serial steps, then aliquots from each dilution were used to seed serial PMCAb reactions. Example of a western blot of serial PMCAb (sPMCAb) products amplified for six rounds is shown in plots a and b . Panel c shows products of PMCAb reactions seeded with four dilutions and amplified for 2, 3 or 6 serial rounds. The dilutions shown for PMCAb reactions were normalized per gram of brain tissue, to correct for differences in assay volumes used for PMCAb (100 μl) and bioassay (50 μl). Full size image In our experience, PMCAb displays a high level of selectivity for infection-specific forms of PrP. To date, we have detected no false-positive amplifications in the routine control reactions that are included with every PMCAb titration experiment. These controls consist of six serial rounds of 48 cycles of PMCAb of unseeded substrate only. Other controls include six rounds of serial PMCAb of 10% normal BHs from 700-day-old hamsters ( Fig. 2 ), and PMCAb amplifications of hamster substrate seeded with full-length recombinant hamster PrP amyloid fibrils prepared under a variety of previously described experimental conditions and protocols [32] , [33] , [34] , [35] . No positive signals were detected in any of the controls ( Fig. 2 ). 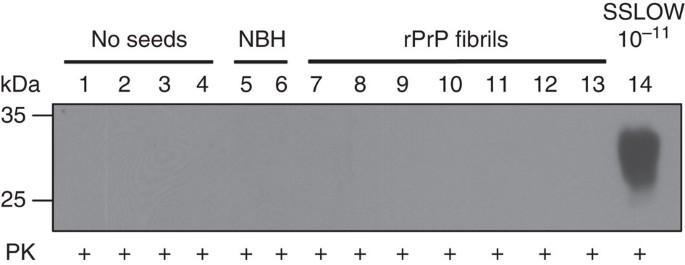Figure 2: Testing the specificity of PrPScdetection in sPMCAb. sPMCAb reactions were seeded with 10% NBH from 700-day-old Syrian hamsters (lanes 5 and 6), recombinant PrP (rPrP) amyloid fibrils type I not subjected to annealing (lane 7); fibrils type I subjected to annealing in Triton (lane 8), BSA (lane 9) or NBH (lanes 10, 11 and 12); with rPrP amyloid fibrils type II (lane 13); or 1011-fold diluted SSLOW brain material (lane14). Four non-seeded reactions are shown in lanes 1, 2, 3 and 4. Six rounds of sPMCAb were conducted for each seeded condition and non-seeded reaction. The final concentration of rPrP amyloid fibrils in serial PMCAb reactions was 10 μg ml−1. rPrP fibrils were prepared using Syrian Hamster full-length rPrP; fibrils type I were prepared in 2M guanidine hydrochloride (GdnHCl) as described by Bocharovaet al.32; fibrils type II were prepared in 0.5 M GdnHCl as described by Sunet al.34rPrP fibrils type I were subjected to annealing in 1% Tritorn X-100, 5 mg ml−1BSA or 5% NBH as described by Bocharovaet al.33and Makaravaet al.31. After six sPMCAb rounds, all samples were treated with PK as described in Methods; western blots were stained with 3F4. To rigorously test the specificity of sPMCAb for detecting PrPSc, multiple experiments were performed using four Misonix S-4000 sonicators over a 2-year period. Several independently prepared stocks of rPrP amyloid fibrils of each type were produced using rPrP from several independent purifications. All results on sPMCAb seeding by rPrP fibrils were negative, confirming that sPMCAb is highly specific for PrPSc. Figure 2: Testing the specificity of PrP Sc detection in sPMCAb. sPMCAb reactions were seeded with 10% NBH from 700-day-old Syrian hamsters (lanes 5 and 6), recombinant PrP (rPrP) amyloid fibrils type I not subjected to annealing (lane 7); fibrils type I subjected to annealing in Triton (lane 8), BSA (lane 9) or NBH (lanes 10, 11 and 12); with rPrP amyloid fibrils type II (lane 13); or 10 11 -fold diluted SSLOW brain material (lane14). Four non-seeded reactions are shown in lanes 1, 2, 3 and 4. Six rounds of sPMCAb were conducted for each seeded condition and non-seeded reaction. The final concentration of rPrP amyloid fibrils in serial PMCAb reactions was 10 μg ml −1 . rPrP fibrils were prepared using Syrian Hamster full-length rPrP; fibrils type I were prepared in 2M guanidine hydrochloride (GdnHCl) as described by Bocharova et al . [32] ; fibrils type II were prepared in 0.5 M GdnHCl as described by Sun et al . [34] rPrP fibrils type I were subjected to annealing in 1% Tritorn X-100, 5 mg ml −1 BSA or 5% NBH as described by Bocharova et al . [33] and Makarava et al . [31] . After six sPMCAb rounds, all samples were treated with PK as described in Methods; western blots were stained with 3F4. To rigorously test the specificity of sPMCAb for detecting PrP Sc , multiple experiments were performed using four Misonix S-4000 sonicators over a 2-year period. Several independently prepared stocks of rPrP amyloid fibrils of each type were produced using rPrP from several independent purifications. All results on sPMCAb seeding by rPrP fibrils were negative, confirming that sPMCAb is highly specific for PrP Sc . Full size image End-point dilution titration in animals In parallel to PMCAb titration, the infectivity titres of brains from 263K- and SSLOW-infected animals were measured using end-point dilution bioassay. Animals were considered infected if they develop symptomatic disease or if their brains contained PrP Sc , as judged by western blot even without symptomatic disease. The fractions of animals infected at each dilution are presented in Table 1 . Table 1 Summary of end-point titration of 263K and SSLOW. Full size table Analysis of prion titre For each dilution, the fraction of animals infected or the fraction of PMCAb reactions with a positive signal on western blot was plotted against the logarithm of dilution for both 263K and SSLOW ( Fig. 3 ). At limiting dilution, PrP Sc particles must necessarily assort randomly into the reaction aliquots, and their distribution is described by the Poisson equation. While there was a good fit to the Poisson equation by the animal infectivity data for both 263K and SSLOW, the PMCAb titration curves for both strains showed a more gradual slope than predicted by the Poisson equation ( Fig. 3a ). This is consistent with increasing reaction efficiency at higher dilutions. One possibility is that dilution results in a concentration-dependent dissociation of aggregates, thereby releasing and increasing the concentration of PMCAb reactive centres. Alternatively, dilution might diminish the effects of an inhibitor. As the effect is at very high dilutions, the inhibitor alternative seems less likely. 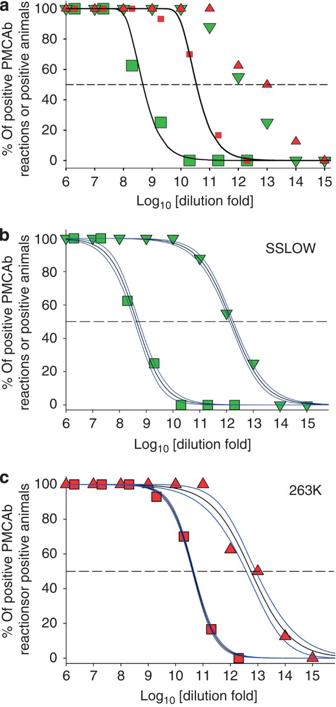Figure 3: Correlation of prion infectivity titre by end-point titration bioassay with PMCAb activity. Brain homogenate materials from Syrian Hamsters infected with SSLOW (large green symbols) or 263K (small red symbols) were subjected to ten-fold serial dilution, then each dilution was analysed by animal bioassay or serial PMCAb. Percentage of animals infected (squares) or giving positive PMCAb reactions (triangles) is plotted as a function of dilution. (a) Analysis of the data using the Poisson function, where the solid curves represent the results of nonlinear least-square best fit. Analysis of the data for SSLOW (b) or 263K (c) using a sigmoidal function. The solid curves represent the results of a nonlinear least-squares best fit and the blue curves represent 95% confidence intervals. ID50and PMCAb50values were calculated from the results of fitting. Figure 3: Correlation of prion infectivity titre by end-point titration bioassay with PMCAb activity. Brain homogenate materials from Syrian Hamsters infected with SSLOW (large green symbols) or 263K (small red symbols) were subjected to ten-fold serial dilution, then each dilution was analysed by animal bioassay or serial PMCAb. Percentage of animals infected (squares) or giving positive PMCAb reactions (triangles) is plotted as a function of dilution. ( a ) Analysis of the data using the Poisson function, where the solid curves represent the results of nonlinear least-square best fit. Analysis of the data for SSLOW ( b ) or 263K ( c ) using a sigmoidal function. The solid curves represent the results of a nonlinear least-squares best fit and the blue curves represent 95% confidence intervals. ID 50 and PMCAb 50 values were calculated from the results of fitting. Full size image An arbitrary sigmoidal function and nonlinear regression analysis were used to calculate ID 50 or PMCAb 50 values from bioassay- or PMCAb-based end-point curves, respectively ( Fig. 3b,c , Table 2 ). (Note that the Poisson equation is a special instance of the more generalized sigmoidal function used.) The infectivity titres determined in this way were almost identical to those determined by the Poisson equation or by more traditional application of the Reed and Meunch and Spearman and Karber methods ( Table 2 ). Analogous to the bioassay, a PMCAb 50 is the reciprocal of the concentration at which only 50% of the PMCAb reactions were positive. As judged from ID 50 and PMCAb 50 values, PMCAb was more sensitive than bioassay by ∼ 4,000-fold for SSLOW and ∼ 160-fold in the case of 263K. Importantly, PMCAb titration was completed in a few days, whereas the bioassay required nearly 2 years. Table 2 ID 50 values measured by end-point bioassay or PMCAb. Full size table We show here that PMCAb, when well calibrated against bioassay, can be used to obtain an estimate of PrP Sc titre in only 3–6 days, ∼ 100 times faster than the bioassay. At the same time, PMCAb offers ethical advantages of reducing the need for animal use. The precision of the measurements in PMCAb is limited only by the number of replicates performed. The new PMCAb-based assay can be used as a fast, efficient and ultrasensitive method for determining PrP Sc titre and is uniquely beneficial for samples that have extremely low levels of infectivity and for determining infectivity concentrations for prion strains with long incubation times. On the other hand, while PMCA has been used for amplification of PrP Sc from a wide range of species [16] , [18] , [19] , [20] , [21] , [22] , [23] , [24] , [25] , the most robust amplification was achieved, so far, for a limited number of rodent or rodent-adapted strains. Further technical improvements are needed for PMCA to be used as a platform for quantitative estimates of PrP Sc from a broad range of species. In recent studies, Soto and co-workers [16] estimated the amount of PrP Sc based on the number of PMCA rounds necessary to amplify prions to a detectible level. While PMCAb and PMCA methods have similar sensitivities for detection of 263K, PMCA requires 18 days to reach sensitivity comparable with that achieved by PMCAb in 3 days. Furthermore, PMCA did not work well for amplification of SSLOW PrP Sc (ref. 29 ). PMCAb is also far less sensitive to inhibitors and small variations in sonication conditions that have plagued conventional PMCA. It is of interest to consider the molecular relationship of PMCAb titre to prion infectivity. A PMCAb 50 titre represents the number of PMCAb-active, PrP Sc -particles capable of initiating PMCAb amplification per gram of material sampled. Both PMCAb amplification products and PrP Sc are heterogeneous in at least size, and perhaps structure, and exactly which structures represent infectivity is not yet clear. Furthermore, contradictory data exist regarding the specific infectivity of PMCA-generated versus that of brain-derived PrP Sc (refs 36 , 37 ). Close comparison of the two sets of data, obtained from the end-point dilution titration on animals and PMCAb, can be used to establish a quantitative relationship. The ratio of PMCAb 50 /ID 50 is the number of PMCAb-active particles that corresponds to one prion infectious dose or unit. The PMCAb 50 /ID 50 ratio was 160 and 4,000 particles per one infectious dose for 263K and SSLOW, respectively ( Table 2 ). There are several ways to explain the 10 2 - to 10 3 -fold excess in the number of PMCAb-active particles over the number of the infectious doses. The large PMCAb 50 /ID 50 ratio could be interpreted as only a few or one out of each 160 or 4,000 PrP Sc particles being truly infectious, whereas the majority of particles while detectible and amplifiable by PMCAb have little or no infectivity. Consistent with this interpretation, recent studies reported a dissociation between PMCA seeding ability and biological infectivity for PrP Sc seeds produced from PrP constructs with deletions of polybasic domains [38] . Furthermore, the studies by Klingeborn et al . [36] showed that PrP Sc generated in PMCA had considerably lower infectivity titre than that of brain-derived PrP Sc (ref. 36 ). This work suggested that two competitive PMCA pathways that amplify infectious PrP Sc and non-infectious particles exist. In contrast, the work by Shikiya and Bartz [37] reported that PMCA-generated PrP Sc had a titre similar to that of brain-derived PrP Sc . Further studies are needed to clarify these contradictory results. Alternatively, the differences between ID 50 and PMCAb 50 values might reflect substantial differences in obstacles to successfully initiate prion infection in an animal versus PMCAb reaction. It has been reported that prions inoculated into animals are subject to intensive proteolytic degradation and clearance [39] . In contrast, the PMCAb amplification is conducted in the presence of protease inhibitors to prevent degradation of the normal prion protein substrate for conversion. It is conceivable that this environment also preserves a greater fraction of infectious PMCAb-active particles, thereby accounting for the ∼ 10 2 - to 10 3 -fold greater sensitivity of the PMCAb assay. Strain 263K (short incubation, short clinical duration) and SSLOW (very long incubation and clinical duration [31] ) represent the two extremes of prion hamster disease. Nevertheless, the concentration of PMCAb-reactive particles was similar in brains of animals infected with 263K or SSLOW ( Table 2 ). No PMCAb-reactive particles were found in brains from aged animals, confirming that these particles are disease-specific. In contrast to having similar PMCAb 50 values, the infectivity titre was ∼ 100-fold lower for SSLOW than for 263K ( Table 2 ). The PMCAb 50 /ID 50 ratio was 160 and 4,000 particles for 263K and SSLOW, respectively ( Table 2 ). If the hypothesis that PMCAb amplifies infectious and non-infectious prion protein seeds is correct, then PMCAb 50 /ID 50 value reflects a strain-specific ratio of non-infectious, disease-associated PMCAb-reactive particles per infectious PrP Sc seeds. Alternatively, the difference in the PMCAb 50 /ID 50 ratio could also reflect strain-specific differences in the amount of PMCAb-active particles required to infect an animal. The difference in efficiency of infection between the two strains could be attributed to several factors. First, the differences could be due to the differences in strain-specific rates of PrP Sc clearance on inoculation. Second, the PrP Sc species that is the most reactive in PMCAb might be not the one that is the most toxic. In fact, previous studies pointed to an uncoupling of prion infectious titre and neurotoxicity [40] . While PMCAb presumably counts PrP Sc particles, the read-out parameter for bioassay is the presence of clinical or subclinical disease, which results from an accumulation of neurotoxic PrP species. Therefore, if infectious and neurotoxic PrP species are two different entities, the differences in PMCAb 50 /ID 50 value could reflect a complex strain-specific relationship between a PMCAb-active PrP Sc species and a neurotoxic species. The strain-specific difference in the PMCAb 50 /ID 50 ratio was mainly due to the substantially lower ID 50 titre of SSLOW in comparison with that of 263K. We do not know whether we would have eventually seen an ID 50 for SSLOW equivalent to that of 263K, if hamsters had longer lifespans in which to develop infections from low titre inocula. In this respect, PMCAb offers advantages over the bioassay for titering slow prion strains, as the read-out parameter in PMCAb is not limited by the lifespan of an animal. Further comparison of end-point titration data from bioassay and PMCAb will test whether PMCAb 50 /ID 50 ratio represents an inherent strain-specific property. Fortunately, uncertainties as to the relationship of PMCAb-active particles to infectivity do not diminish the power or usefulness of PMCAb as a quantitative assay. PMCAb can be used as is, as a relative indicator of infectivity titre between two similar samples. With careful calibration and sample control, it can be used to estimate PrP Sc infectivity titre itself. End-point titration bioassay This study was carried out in strict accordance with the recommendations in the Guide for the Care and Use of Laboratory Animals of the National Institutes of Health. The protocol was approved by the Institutional Animal Care and Use Committee of the University of Maryland, Baltimore (assurance number: A32000-01; permit number: 0309001). Ten percent scrapie BH was prepared in PBS, pH 7.4, by sonication and serially diluted up to 10 11 -fold in PBS, as previously described [41] . SSLOW-inoculated animals from the second passage of SSLOW [31] were used for both bioassay and PMCAb. Before inoculation, samples were dispersed by 90 s of maximum power ultrasonication in PBS. Each hamster received 50-μl inoculum intracerebrally under general anaesthesia (2 LPM O 2 /4 MAC isoflurane). The inoculated animals were observed closely for up to 660 days post-inoculation or until they developed clinical signs of prion disease. For SSLOW-inoculated animals, the clinical signs were observed as early as 318±10 days post-inoculation for the 10-fold dilution of brain material or as late as 560±10 days for the 10 6 -fold dilution of brain material. Only one out of eight animals inoculated with the 10 7 -fold dilution showed clinical signs, whereas no clinical signs were observed for dilutions 10 8 -fold and higher. Affected animals were euthanized and their disease status was confirmed by western blot analysis of their brains. At the end of the incubation (660 days post-inoculation) all remaining animals were euthanized, and all brains were assessed for the presence of PrP Sc by western blot. Animal brains that contained PrP Sc but had not yet developed symptomatic disease were considered infected. End-point titration using PMCAb Healthy hamsters were euthanized and immediately perfused with PBS, pH 7.4, supplemented with 5 mM EDTA. Brains were dissected, and 10% BH (wt/vol) was prepared using ice-cold conversion buffer and glass/Teflon tissue grinders cooled on ice and attached to a constant torque homogenizer (Heidolph, RZR2020). The brains were ground at low speed until homogeneous, and then five additional strokes completed the homogenization. The composition of conversion buffer was as previously described [11] : Ca 2+ -free and Mg 2+ -free PBS, pH 7.4, supplemented with 0.15 M NaCl, 1.0% Triton and 1 tablet of Complete protease inhibitors cocktail (Roche, cat. no. 1836145) per 50 ml of conversion buffer. The resulting 10% normal BH (NBH) in conversion buffer was used as the substrate in PMCA reactions. To prepare seeds, scrapie-infected brains were homogenized as for inoculation (above), and 100 μl aliquots were sonicated in MISONIX S-400 microplate (Misonix) horn for 30 s at 50% power before serial dilution from 10- to 10 14 -fold in conversion buffer. Then, 10 μl of each dilution were used to seed 90 μl of NBH for PMCAb. Teflon beads (2.38 mm diameter, McMaster-Carr, Los Angeles, CA, USA) were placed into the 0.2 ml tubes first, and then NBH and seeds were added. Samples in 0.2 ml thin-wall PCR tubes (Fisher, cat. no. 14230205) were placed in a floating rack inside a Misonix S-4000 microplate cup horn filled with 350 ml water. Two coils of rubber tubing attached to a circulating water bath were installed for maintaining 37 °C inside the sonicator chamber. The standard sonication program consisted of 30 s sonication pulses delivered at 50% efficiency applied every 30 min during a 24-h period. For each subsequent round of serial PMCAb, 10 μl aliquotes from a previous round were used to seed the reactions in the next round. At limiting dilutions, up to ten independent serial PMCAb reactions were used for each dilution to accumulate statistics. Data analysis To correct for differences in assay volumes used for PMCAb (100 μl) and bioassay (50 μl), the fraction of positive PMCAb reactions or positive animals, presented in Fig. 3 , were normalized per gram of brain tissue. Analysis using Poisson equation For the probability that a given aliquot received no active particle, P (0), the Poisson equation reduces to P (0)=e − m , where m is the concentration of the active particle at that dilution in particles per inoculation volume. The probability that there will be at least one active particle to initiate infection, P (≥1), is P (≥1)=1−e − m . The infectivity data were fit to the expression: where F is fraction of infected animals, x is dilution and a is the fitted parameter equal to the undiluted concentration of infectivity. ID 50 was calculated by solving the fitted equations for F =0.5 (infectivity), which reduce to the expression: Analysis using sigmoidal equation ID 50 and PMCAb 50 values were determined by regression analysis in Sigma Plot using nonlinear least squares fitting of both sets of data to the sigmoidal equation: where F is percent of positive PMCAb reactions or infected animals, x is logarithm of the dilution fold, A and B are two fitting parameters that define the position of a limiting dilution transition on the x axis and the slope of the transition, respectively. ID 50 and PMCAb 50 were calculated according to the equation: Proteinase K assay To analyse the PMCAb end-point titration reactions, 10 μl of each sample was supplemented with 5 μl SDS and 5 μl proteinase K (PK), to a final concentration of SDS and PK of 0.25% and 50 μg ml -1 , respectively, followed by incubation at 37°C for 1 h. The digestion was terminated by addition of SDS sample buffer and boiling for 10 min. Samples were loaded onto NuPAGE 12% BisTris gels, transferred to polyvinylidene difluoride membrane, and stained with 3F4 antibody. To analyse scrapie BHs, an aliquot of 10% BH was mixed with an equal volume of 4% sarcosyl in PBS, supplemented with 50 mM Tris, pH 7.5, and digested with 20 μg ml −1 PK for 30 min at 37°C with 1,000 r.p.m. shaking (Eppendorf Thermomixer). The reaction was stopped by SDS sample buffer. Samples were boiled for 10 min and loaded onto NuPAGE 12% BisTris gels. After transfer to polyvinylidene difluoride membrane, PrP was detected with 3F4 antibody. How to cite this article: Makarava, N. et al . Fast and ultrasensitive method for quantitating prion infectivity titre. Nat. Commun. 3:741 doi: 10.1038/ncomms1730 (2012).